Corals concentrate dissolved inorganic carbon to facilitate calcification The sources of dissolved inorganic carbon (DIC) used to produce scleractinian coral skeletons are not understood. Yet this knowledge is essential for understanding coral biomineralization and assessing the potential impacts of ocean acidification on coral reefs. Here we use skeletal boron geochemistry to reconstruct the DIC chemistry of the fluid used for coral calcification. We show that corals concentrate DIC at the calcification site substantially above seawater values and that bicarbonate contributes a significant amount of the DIC pool used to build the skeleton. Corals actively increase the pH of the calcification fluid, decreasing the proportion of DIC present as CO 2 and creating a diffusion gradient favouring the transport of molecular CO 2 from the overlying coral tissue into the calcification site. Coupling the increases in calcification fluid pH and [DIC] yields high calcification fluid [CO 3 2− ] and induces high aragonite saturation states, favourable to the precipitation of the skeleton. Neither the sources [1] nor the species [2] , [3] of dissolved inorganic carbon (DIC) used during coral calcification are understood. The aragonite skeleton precipitates from an extracellular calcification fluid (ECF) enclosed in a semi-isolated space between the skeleton and the overlying coral tissue. The DIC utilized to form the coral skeleton is derived from seawater and from an internal DIC pool [1] , [4] . An active bicarbonate transporter has not been ruled out in coral, but dual-radiolabelling studies suggest that this is not the source of additional carbon [4] . The isotopically light carbon and oxygen compositions of coral skeletons suggest that molecular CO 2 may act as the source of internal DIC [5] . Understanding the sources of skeletal carbon is key to the accurate prediction of the effects of increasing [DIC] in seawater (ocean acidification) and for the correct interpretation of δ 18 O and δ 13 C coral-based palaeoenvironmental records. We analysed the B/Ca and B isotope ratios (δ 11 B) of coral aragonite to reconstruct the DIC chemistry of the coral ECF. Dissolved boron in seawater occurs primarily as boric acid, B(OH) 3 , and borate, B(OH) 4 − , and speciation is controlled by ambient pH [6] . Borate is selectively incorporated into aragonite [7] , presumably substituting for CO 3 2− in the lattice. There are no known active transport mechanisms for boron in corals and we assume that dissolved boron is transported to the ECF in seawater. Seawater transport to the ECF is a passive process [8] and as such the transport rate is likely to be constant. At equilibrium, B(OH) 3 is enriched in 11 B compared with B(OH) 4 − (ref. 9 ), hence the δ 11 B of coral aragonite reflects ECF pH. Skeletal [B] reflects both ECF pH and the concentration of the DIC species competing with borate for inclusion in the carbonate [10] . Passive diffusion of B(OH) 3 across cell membranes [11] could potentially offset ECF δ 11 B from seawater values. However, ECF pH estimates derived from skeletal δ 11 B compare well with direct characterizations using fluorescent probes, suggesting that this effect is insignificant, that is, the observed ECF pH in Stylophora pistillata (8.69 and 8.36 in the light and dark, respectively) cultured at seawater pH 8.1 (ref. 12 ) is in excellent agreement with δ 11 B of the same species cultured at pH 8.09 (24.8‰, equivalent to an ECF pH of 8.55) [13] , assuming that calcification is three times faster in the light than in the dark [14] . A recent suggestion that skeletal δ 11 B ECF pH estimates may be offset to lower values than expected [15] is based on a comparison of skeletal δ 11 B and direct ECF pH measurements in the light only. ECF pH is lower in the dark [16] and this likely accounts for the offset. We used skeletal δ 11 B to estimate ECF pH [17] and B/Ca to estimate the concentration of the DIC species that co-precipitates with B(OH) 4 − . It is not clear whether CO 3 2− or HCO 3 − ions are utilized during coral aragonite precipitation [2] , [3] . We consider three scenarios: that B(OH) 4 − co-precipitates with CO 3 2− only (scenario 1), with HCO 3 − only (scenario 2) or with both CO 3 2− and HCO 3 − (scenario 3). We estimated the B(OH) 4 − /CO 3 2− , B(OH) 4 − /HCO 3 − and B(OH) 4 − /(CO 3 2− +HCO 3 − ) aragonite partition coefficients from an estimate of the δ 11 B and B/Ca of secondary aragonite cement in a fossil coral coupled with alkalinity measurements of coral skeletal pore fluids [18] . We used our estimates of ECF pH and co-precipitating DIC species to calculate the concentrations of the other carbonate system variables in the ECF, namely, all other DIC species and total alkalinity (TA). We show that the ECF pH and DIC chemistry are significantly different from that of seawater and that bicarbonate contributes a significant amount of the DIC pool used to build the skeleton. Modern Porites spp. field corals We analysed three modern massive Porites spp. field corals from Oahu, Hawaii, and Jarvis Island, South Pacific. Skeletal δ 11 B ECF pH estimates ( Fig. 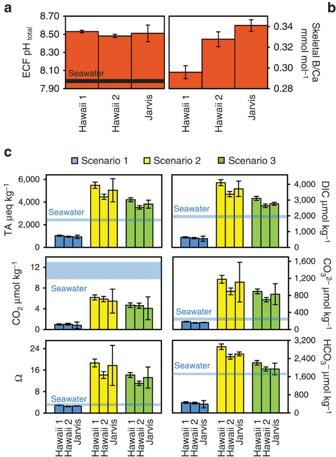Figure 1: Geochemistry and reconstructed calcification fluid DIC ofPoritesspp. field corals. (a) ECF pH (from skeletal δ11B), (b) skeletal B/Ca and (c) reconstructed ECF DIC system parameters. Ω, aragonite saturation state. Both δ11B and B/Ca are normally distributed in each coral and error bars are 95% confidence limits (s.e.m.). Data are means of ≥99 B/Ca analyses and ≥40 δ11B analyses with the exception of δ11B in the Jarvis coral where only 12 analyses were made, note the larger confidence limits. DIC system errors are calculated from propagating 95% confidence limits in B/Ca and δ11B analyses onto DIC system estimates. Horizontal lines denote seawater concentrations and are calculated from observations of pH and TA in Jarvis Island benthic reefwater29and DIC and TA in Hawaii reefwater33. 1 ; Table 1 ) confirm that corals actively increase the pH of the ECF above that of seawater [12] , [16] . The ECF composition reflects the balance of DIC inputs and outputs, namely, seawater diffusion, molecular CO 2 invasion, proton extrusion and calcification ( Fig. 2 ). CO 2 invasion does not influence TA and the departure of ECF [TA] from seawater values reflects calcification (reduces [TA]) and proton extrusion (increases [TA]). Similarly, proton extrusion does not affect [DIC] and the departure of ECF [DIC] from seawater values reflects calcification (reduces [DIC]) and CO 2 invasion (increases [DIC]). Figure 1: Geochemistry and reconstructed calcification fluid DIC of Porites spp. field corals. ( a ) ECF pH (from skeletal δ 11 B), ( b ) skeletal B/Ca and ( c ) reconstructed ECF DIC system parameters. Ω, aragonite saturation state. Both δ 11 B and B/Ca are normally distributed in each coral and error bars are 95% confidence limits (s.e.m.). Data are means of ≥99 B/Ca analyses and ≥40 δ 11 B analyses with the exception of δ 11 B in the Jarvis coral where only 12 analyses were made, note the larger confidence limits. DIC system errors are calculated from propagating 95% confidence limits in B/Ca and δ 11 B analyses onto DIC system estimates. Horizontal lines denote seawater concentrations and are calculated from observations of pH and TA in Jarvis Island benthic reefwater [29] and DIC and TA in Hawaii reefwater [33] . Full size image Table 1 Measured B/Ca and δ 11 B in each coral colony and ECF pH estimated from δ 11 B. 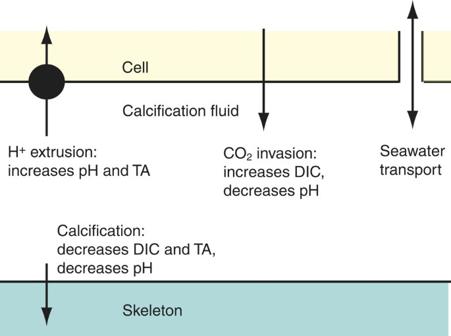Figure 2: Schematic of the processes affecting the DIC system in the coral calcification fluid. The DIC composition reflects the balance of inputs and outputs, namely, seawater diffusion, molecular CO2invasion, proton extrusion and calcification. Full size table Figure 2: Schematic of the processes affecting the DIC system in the coral calcification fluid. The DIC composition reflects the balance of inputs and outputs, namely, seawater diffusion, molecular CO 2 invasion, proton extrusion and calcification. Full size image Under scenario 1 (borate co-precipitates with CO 3 2− ), the ECF has [DIC] and [TA], which are substantially lower than ambient seawater ( Fig. 1 ). Ca-ATPase activity has little effect on the [Ca] of the ECF [19] and in scenario 1, the aragonite saturation state (Ω) of the ECF (essentially a product of [Ca] and [CO 3 2− ]) is ~3 and below that of seawater (Ω=~4). It is implausible that the high calcification rates observed in tropical corals are attained with such an impoverished ECF and we reject this scenario. Scenario 2 (borate co-precipitates with HCO 3 − ) and scenario 3 (borate co-precipitates with both HCO 3 − and CO 3 2− ) produce broadly similar results ( Fig. 1 ), as HCO 3 − is the most abundant carbon species (70–90%) over the observed ECF pH range. Proton pumping maintains ECF TA in the untreated corals well above seawater concentrations and [DIC] is up to double that of ambient seawater ( Fig. 1 ). ECF Ω in the untreated corals rises to 11–19, depending on coral and scenario, and facilitates rapid aragonite precipitation. These are both credible scenarios. Our observation that borate co-precipitates with HCO 3 − in the aragonite lattice indicates that a large proportion of skeletal carbon is ultimately derived from the bicarbonate of the ECF. It is unknown whether HCO 3 − deprotonates before or after binding to the aragonite [20] , but the key point is that bicarbonate contributes to the DIC pool used during calcification. Under scenarios 2 and 3, up to half of the DIC used in calcification does not come though the seawater transport pathway. The enzyme-driven increase in ECF pH shifts the DIC equilibrium in favour of CO 3 2− at the expense of CO 2 and HCO 3 − , creating a diffusion gradient favouring the diffusion of molecular CO 2 from the overlying coral tissue into the ECF [21] . We conclude that this is a likely source of the additional skeletal carbon. This interpretation is supported by geochemical and modelling studies, which indicate that a substantial proportion of coral aragonite is derived from an isotopically light (with respect to carbon and oxygen) molecular CO 2 source [5] , [21] . We note that ECF [CO 2 ] in the field corals is significantly below that of seawater. Either CO 2 diffusion rate into the ECF is rate limited or the mean [CO 2 ] in the overlying coral tissue is reduced below that of seawater. Cultured Pocillopora damicornis To investigate this further, we analysed cultured colonies of the branching coral, Pocillopora damicornis , some of which were incubated with the Ca-ATPase enzyme inhibitor, ruthenium red [22] . Ca-ATPase pumps Ca 2+ into and H + out of the ECF and increases ECF pH [19] . Ruthenium red solutions absorb light from 430 to 615 nm; however, the collective evidence suggests that the chemical reduces coral calcification rate by directly inhibiting Ca-ATPase rather than by inhibiting zooxanthellar photosynthesis [22] . This experiment was designed to explore the response of ECF DIC chemistry to changes in ECF pH and all the cultured colonies were grown (by asexual budding and division) from branches of a single-parent colony, that is, all colonies were genetically identical. We do not infer that the ECF DIC chemistry of the cultured colonies is representative of this coral species in the field. We cultured duplicate corals in each treatment and in the solvent control and a single colony in the seawater control. We model the ECF DIC chemistry for each coral colony separately ( Fig. 3 ). Inhibition of Ca-ATPase decreased skeletal δ 11 B (and ECF pH) in the high ruthenium red treatment compared with both the seawater and the dimethyl sulfoxide (DMSO) controls. 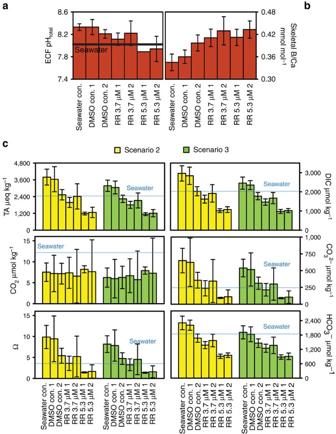Figure 3: Geochemistry and reconstructed calcification fluid DIC of culturedP. damicorniscorals. (a) ECF pH (from skeletal δ11B), (b) skeletal B/Ca and (c) reconstructed ECF DIC system parameters. Ω, aragonite saturation state. Error bars are 95% confidence limits (s.e.m.). Cultured corals were exposed to ruthenium red (RR) dissolved in 0.1% DMSO and DMSO and seawater-only controls (con.) were also analysed. Corals were analysed in duplicate (indicated by 1 or 2 annotation). Analyses (7–16) were collected on each sample (Table 1) with the exceptions of RR 3.7 μM 2 and RR 5.3 μM 1 where only 2 and 1, respectively, credible δ11B analysis (exhibiting the42Ca spike throughout the analysis) were obtained. Errors are calculated as for the field corals and horizontal lines denote seawater concentrations calculated from observations of pH and TA in the culture seawater22. Figure 3: Geochemistry and reconstructed calcification fluid DIC of cultured P. damicornis corals. ( a ) ECF pH (from skeletal δ 11 B), ( b ) skeletal B/Ca and ( c ) reconstructed ECF DIC system parameters. Ω, aragonite saturation state. Error bars are 95% confidence limits (s.e.m.). Cultured corals were exposed to ruthenium red (RR) dissolved in 0.1% DMSO and DMSO and seawater-only controls (con.) were also analysed. Corals were analysed in duplicate (indicated by 1 or 2 annotation). Analyses (7–16) were collected on each sample ( Table 1 ) with the exceptions of RR 3.7 μM 2 and RR 5.3 μM 1 where only 2 and 1, respectively, credible δ 11 B analysis (exhibiting the 42 Ca spike throughout the analysis) were obtained. Errors are calculated as for the field corals and horizontal lines denote seawater concentrations calculated from observations of pH and TA in the culture seawater [22] . Full size image However, there is little variation in reconstructed ECF [CO 2 ] despite the large ECF pH range observed in these specimens. To illustrate the relationships between ECF pH and DIC chemistry, we plotted ECF [DIC] and Ω as a function of ECF pH and CO 2 assuming that CO 2 diffuses freely into the ECF maintaining equilibrium with an overlying CO 2 source ( Fig. 4 ). ECF DIC increases with increasing pH, reflecting the conversion of CO 2 to other DIC species at high pH and the diffusion of additional CO 2 into the ECF, thereby concentrating DIC. Ω increases with increasing pH, reflecting the increase in ECF [CO 3 2− ] with pH. The data sets from both the cultured and field corals indicate that ECF [CO 2 ] is approximately a third to a half of that in ambient seawater across all treatments. We are unable to determine whether this reflects an equilibrium with the overlying CO 2 source or indicates a rate limitation on the diffusion of CO 2 into the ECF. We find a strong positive correlation between ECF aragonite saturation state and coral calcification rate ( Fig. 5 ), although we note that the rate dependence in coral is less than that in aragonite inorganically precipitated at the same temperature, that is, doubling aragonite saturation state increases precipitation by 1.5 × in coral and 5 × in synthetic aragonite [23] . This is perhaps to be expected. Corals do not precipitate randomly but exert exquisite control over both the sites of precipitation and the crystal morphology [24] . 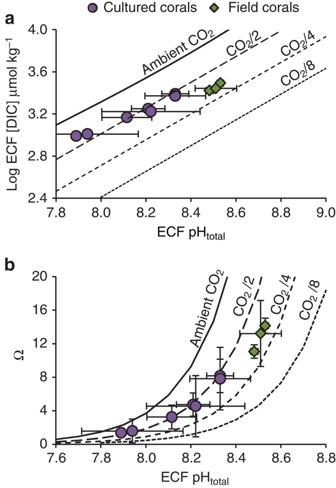Figure 4: Modelled relationships between calcification fluid pH and DIC parameters. The relationships were modelled under a range of CO2scenarios. (a) ECF [DIC] and (b) ECF aragonite saturation state (Ω) increase with ECF pH, assuming that CO2readily diffuses into the calcification site, maintaining an equilibrium with an overlying [CO2] ranging from that of ambient seawater to 1/8 of this. DIC calculations were made using CO2sys30, assuming seawaterT=25 °C andS=40.6, that is, the conditions in the culture seawater. Reconstructed DIC parameters under scenario 3 in the field and cultured corals are overlain on each graph. Field corals grew under different temperatures and salinities, but this does not affect the interpretation of these graphs. Error bars are 95% confidence limits (s.e.m.) and in the case of ECF DIC are smaller than the heights of the symbols. Figure 4: Modelled relationships between calcification fluid pH and DIC parameters. The relationships were modelled under a range of CO 2 scenarios. ( a ) ECF [DIC] and ( b ) ECF aragonite saturation state (Ω) increase with ECF pH, assuming that CO 2 readily diffuses into the calcification site, maintaining an equilibrium with an overlying [CO 2 ] ranging from that of ambient seawater to 1/8 of this. DIC calculations were made using CO 2 sys [30] , assuming seawater T =25 °C and S =40.6, that is, the conditions in the culture seawater. Reconstructed DIC parameters under scenario 3 in the field and cultured corals are overlain on each graph. Field corals grew under different temperatures and salinities, but this does not affect the interpretation of these graphs. Error bars are 95% confidence limits (s.e.m.) and in the case of ECF DIC are smaller than the heights of the symbols. 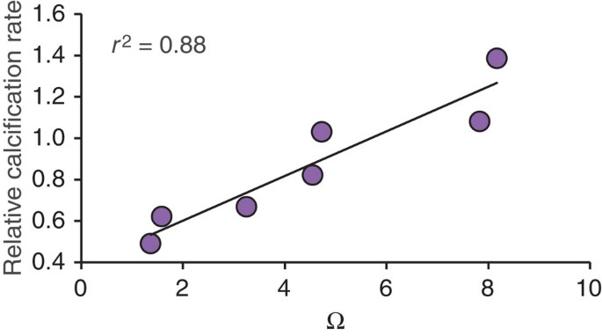Figure 5: Correlation between calcification fluid aragonite saturation state and calcification rate in the cultured corals. Reconstructed calcification fluid aragonite saturation state (Ω) was calculated under scenario 3. Colony calcification rate is calculated from the mean calcification rate measured in the presence of the inhibitor, if used, as a proportion of the calcification rate observed on day 1, before the introduction of the inhibitor22. Full size image Figure 5: Correlation between calcification fluid aragonite saturation state and calcification rate in the cultured corals. Reconstructed calcification fluid aragonite saturation state (Ω) was calculated under scenario 3. Colony calcification rate is calculated from the mean calcification rate measured in the presence of the inhibitor, if used, as a proportion of the calcification rate observed on day 1, before the introduction of the inhibitor [22] . Full size image Our findings have implications for predicting the effects of ocean acidification on coral reefs. Although the ECF pH gradient facilitates the diffusion of CO 2 into the calcification site, we find that ECF [CO 2 ] in all field corals is significantly below that of seawater. Ocean acidification decreases seawater pH but increases seawater [DIC] and [CO 2 ]. Understanding how these changes will impact both ECF pH and the diffusion of CO 2 into the coral ECF as a carbon concentration mechanism is key to interpreting current ocean acidification studies and predicting the effects of future scenarios. Sample processing For further details of field sites and coral-culturing procedures, see refs 17 , 22 , 25 , 26 . Cultured corals were originally collected from the Gulf of Eilat, and were maintained in seawater at ambient salinity (40.6). Each culture experiment lasted for 5 days. Individual colonies were placed in flow-through coral chambers at the start of day 1 and ruthenium red dissolved in DMSO solution to a final concentration of 0.1% DMSO was added to the seawater supplied to the chambers at the start of day 2. A stable isotope tracer ( 42 Ca as 42 CaCO 3 ) was added to the seawater at the same time as the inhibitor, allowing accurate identification of skeleton deposited in the presence of the inhibitor (if used) by secondary ion mass spectrometry (SIMS). This tracer increased the seawater 42 Ca/ 44 Ca from 0.31 to ~0.40 and increased the [Ca] of seawater by ~0.2%. A DMSO control (0.1%) and a seawater control (with the addition of 42 CaCO 3 only) were also tested. All treatments were tested in duplicate. Light and dark coral calcification rates were estimated each day [22] using the alkalinity anomaly technique [2] . Modern field and cultured corals were living when collected/sacrificed. Specimens were immersed in 3–4% sodium hypochlorate ( I ) solutions for ≥8 h with intermittent ultrasonic agitation to remove organic contamination, then rinsed repeatedly in distilled water and dried. Skeletal strips were sawn along the maximum growth axis of the field specimens, divided into 10–15 mm lengths and fixed to 25 mm round thin sections. Branch ends of cultured corals were fixed into 25 mm circular epoxy resin blocks (Epofix, Struers). Sections and blocks were polished using silicon carbide papers (up to 4,000 grade, lubricated with water) and polishing alumina (0.05 μm, suspended in water). Multiple SIMS analyses were evenly spaced across 1 year (Jarvis coral) and 2 years (both Hawaiian corals) of skeletal growth in the field corals. Annual growth bands were identified from X-ray radiographs in the Hawaiian corals and from unpublished δ 13 C data, which exhibit a seasonal trend, in the Jarvis coral. No analyses were made in the outermost parts of the field skeletons, which contained the tissue layers of the corals. In the cultured corals, SIMS analyses were sited on the outermost tips of the skeleton. Analyses that did not exhibit enhanced 42 Ca/ 44 Ca throughout the analysis were rejected. Sections were repolished between batches of analyses to expose fresh areas for SIMS. δ 11 B and B/Ca analyses Skeletal δ 11 B and B/Ca were determined by SIMS in the School of GeoSciences at the University of Edinburgh. The high spatial resolution of SIMS (primary beam diameters=25–40 μm) allows the selective analysis of both the primary coral aragonite, avoiding contamination from secondary cements or microboring organisms, and the small skeletal volumes deposited in the culture experiment. δ 11 B in the Hawaiian and cultured corals were analysed with a Cameca 1270, while the Jarvis coral was analysed with a Cameca 4f. One coral (Hawaii 1) had also previously been analysed using the Cameca 4f [17] and there is excellent agreement in standardized δ 11 B estimates between the two instruments (within 0.4‰, equivalent to a pH of 0.03). B/Ca was determined using the Cameca 4f. Cultured coral analyses were normalized to multiple daily analyses of a Porites spp. coral standard (δ 11 B=24.8‰, B/Ca=0.364 mmol mol −1 (ref. 27 )). The s.d. (1 σ ) of bracketed standard analyses ( n =13–19) each day was δ 11 B=1.7‰ and B/Ca=9%. Field coral analyses were normalized to the same Porites spp. standard, but a more homogenous Desmophyllum spp. cold-water coral chip was used to check for instrumental drift within and between days. The s.d. (1 σ ) of bracketed standard analyses ( n =15–27) each day was δ 11 B=1.2‰ and B/Ca=2%. The precision (2 σ ) of the Porites spp. standard in each session was equivalent to ±0.02 pH units and ±3% B/Ca. Estimation of partition coefficients We estimated B(OH) 4 − /CO 3 2− , B(OH) 4 − /HCO 3 − and B(OH) 4 − /(CO 3 2− +HCO 3 − ) aragonite partition coefficients from δ 11 B and B/Ca analyses of secondary aragonite cement in a Hawaiian fossil coral dated to 13.4 ky. We used δ 11 B to estimate coral pore fluid pH and assumed a porewater TA of 2,162±78 μmol kg −1 ( n =4) based on repeat measurements of skeletal pore fluids in a modern coral [18] . Porewater [Ca] is similar to adjacent reefwaters (within 5%) [18] and we assume that porewater [B] is the same as seawater (416 μmol kg −1 ) at the collection site of the fossil coral. We estimated B(OH) 4 − /CO 3 2− , B(OH) 4 − /HCO 3 − and B(OH) 4 − /(CO 3 2− +HCO 3 − ) aragonite partition coefficients to be 0.283, 4.51 and 4.79, all × 10 −3 , respectively ( Supplementary Table 1 ). Calculation of ECF DIC parameters The equilibrium constant, K B , and its p K B value were calculated [28] from the known temperatures and salinity of the field sites and culture seawater. Mean annual salinity and temperature at the Jarvis and Hawaii reef sites are 35.5 and 27.4 °C (ref. 29 ) and 35.0 and 25.0 °C (ref. 17 ), respectively. Salinity and temperature in the culture system were 40.6 and 25.0 °C (ref. 22 ). ECF pH was estimated from skeletal δ 11 B: using the empirically determined α B (=1.0272) [9] and assuming that the δ 11 B ECF is the same as seawater (39.5‰). We assumed that [B] ECF is the same as seawater, that is, where S is the salinity [28] . We used pH ECF to estimate the [B(OH) 4 − ] ECF : B/Ca aragonite equates to B/CO 3 aragonite 2− as Ca and C are equimolar in CaCO 3 . We used [B(OH) 4 − ] ECF , B/Ca aragonite and the relevant B/(co-precipitating DIC species) partition coefficients to estimate the concentration of the DIC species co-precipitating with B(OH) 4 − in the ECF. For example, We used pH ECF and the concentration of the DIC species co-precipitating with B (OH) 4 − in the ECF (that is, [CO 3 2− ] ECF in scenario 1, [HCO 3 − ] ECF in scenario 2 and so on) to estimate all the other parameters in the ECF DIC system. DIC system parameters were calculated using CO 2 sys.xls [30] using acidity constants K 1 and K 2 from Roy et al . [31] and KHSO 4 from Dickson [32] . ECF Ω was calculated using ECF [CO 3 2− ] and assuming that ECF [Ca 2+ ] was similar to seawater [19] . How to cite this article: Allison, N. et al . Corals concentrate dissolved inorganic carbon to facilitate calcification. Nat. Commun. 5:5741 doi: 10.1038/ncomms6741 (2014).